African origin of the malaria parasitePlasmodium vivax Plasmodium vivax is the leading cause of human malaria in Asia and Latin America but is absent from most of central Africa due to the near fixation of a mutation that inhibits the expression of its receptor, the Duffy antigen, on human erythrocytes. The emergence of this protective allele is not understood because P. vivax is believed to have originated in Asia. Here we show, using a non-invasive approach, that wild chimpanzees and gorillas throughout central Africa are endemically infected with parasites that are closely related to human P. vivax . Sequence analyses reveal that ape parasites lack host specificity and are much more diverse than human parasites, which form a monophyletic lineage within the ape parasite radiation. These findings indicate that human P. vivax is of African origin and likely selected for the Duffy-negative mutation. All extant human P. vivax parasites are derived from a single ancestor that escaped out of Africa. Of the five Plasmodium species known to cause malaria in humans, P. vivax is the most widespread [1] . Although highly prevalent in Asia and Latin America, P. vivax is thought to be absent from west and central Africa due to the near fixation of a mutation that causes the Duffy-negative phenotype in indigenous African people [1] , [2] . The Duffy antigen receptor for chemokines (DARC) is used by P. vivax merozoites to invade red blood cells [3] . Since the absence of DARC on the surface of erythrocytes confers protection against P. vivax malaria, this parasite has long been suspected to be the agent that selected for this mutation [2] , [4] , [5] . However, this hypothesis has been difficult to reconcile with the proposed evolutionary origin of P. vivax [6] , [7] , [8] . The closest relative of P. vivax is believed to be P. cynomolgi [9] , which infects macaques. These two parasites form a lineage within a clade comprised of at least seven other Plasmodium species, all of which infect primates found only in Asia. The consensus view has thus been that P. vivax emerged in Southeast Asia following the cross-species transmission of a macaque parasite [6] , [7] , [8] , [9] . Under this scenario, the Duffy-negative mutation prevalent in west central African people was selected by another unidentified pathogen [4] , and its high frequency prevented P. vivax from entering central Africa. Recently, P. vivax -like parasites have been identified in a limited number of African apes [10] , [11] , [12] , [13] and some mosquitoes ( Anopheles species) trapped in their vicinity [13] , [14] . Molecular characterization of these parasites showed that they are very similar to, but apparently distinct from, human P. vivax [13] . These findings raised the possibility that a sylvatic P. vivax reservoir exists in wild-living apes or other African primate species. However, since only very few of these sylvatic parasites have been identified, information concerning their geographic distribution, host species association, prevalence and relationship to human P. vivax is lacking. In fact, most evidence of this natural P. vivax reservoir has come from pets and apes in wildlife rescue centres. Since captive apes can become infected with Plasmodium species that do not normally infect them in their natural habitat [10] , [15] , studies of wild-living populations are essential. African apes are highly endangered and live in remote forest regions, rendering invasive screening for infectious agents both impractical and unethical. As an alternative, we have developed methods that permit the detection and amplification of pathogen-specific nucleic acids from ape faecal DNA [16] , [17] , [18] , [19] . This approach enabled us to trace the origins of human immunodeficiency virus type 1 (HIV-1) to chimpanzees ( Pan troglodytes ) in west central Africa [18] and to identify the precursor of human P. falciparum in western gorillas ( Gorilla gorilla ) [10] . Here, we used a similar approach to investigate the molecular epidemiology of P. vivax infection in wild-living apes. Screening more than 5,000 faecal samples from 78 remote forest sites, we tested ape communities throughout central Africa. Since conventional PCR analysis is error prone and has the potential to confound phylogenetic analyses [10] , parasite sequences were generated using single-genome amplification (SGA), which eliminates Taq polymerase-induced recombination and nucleotide substitutions from finished sequences [20] , [21] . In this study, we show that western ( G. gorilla ) and eastern gorillas ( G. beringei ) and chimpanzees ( P. troglodytes ), but not bonobos ( P. paniscus ), are endemically infected with P. vivax -like parasites, and that infection rates in wild ape communities are similar to those in human populations with stable parasite transmission. Analysing over 2,600 SGA-derived mitochondrial, apicoplast and nuclear sequences, we also show that ape parasites are considerably more diverse than human parasites and do not cluster according to their host species. In contrast, human parasites form a monophyletic lineage that falls within the radiation of the ape parasite sequences. These results indicate that human P. vivax arose from within a Plasmodium species that infect wild-living chimpanzees and gorillas, and that all extant human P. vivax parasites evolved from a single ancestor that spread out of Africa. Host species association and distribution of ape P. vivax Using PCR primers designed to amplify P. vivax mitochondrial (mt) DNA, we screened 5,469 faecal specimens from ape communities sampled at 78 forest sites throughout sub-Saharan Africa ( Fig. 1 ). 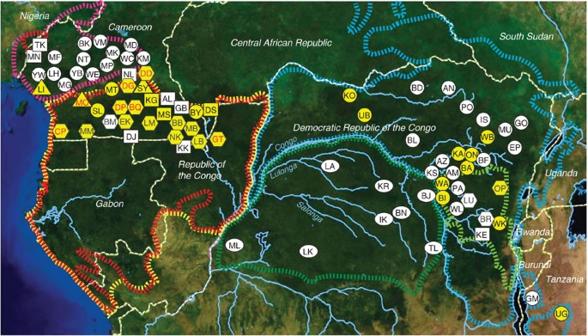Figure 1: Geographic distribution ofP. vivaxin wild-living apes. Field sites are shown in relation to the ranges of three subspecies of the common chimpanzee (P. t. ellioti,magenta;P. t. troglodytes, red; andP. t. schweinfurthii, blue), western (G. gorilla, yellow) and eastern (G. beringei, light green) gorillas, as well as bonobos (P. paniscus, green). Circles, squares and hexagons identify field sites where wild-living chimpanzees, gorillas or both species were sampled, respectively. Ovals indicate bonobo sampling sites. Triangles denote the location of wildlife rescue centres (seeSupplementary Table 1for a list of all field sites and their two-letter codes). Forested areas are shown in dark green, while arid and semiarid areas are depicted in yellow and brown, respectively. Major lakes and major rivers are shown in blue. Dashed white lines indicate national boundaries. Sites where apeP. vivaxwas detected are highlighted in yellow, with red lettering indicating that both chimpanzees and gorillas were infected. Except for 196 samples from habituated apes, all other specimens were derived from non-habituated communities ( Supplementary Table 1 ). Ape species and subspecies were identified by faecal mtDNA analysis [10] , [18] , [19] . A subset of specimens was also subjected to microsatellite analyses to estimate the number of sampled individuals ( Supplementary Table 1 ). Targeting a 297-base-pair (bp) mtDNA fragment ( Supplementary Fig. 1a ), we found P. vivax- like sequences in faecal DNA from western gorillas ( G. gorilla ), eastern gorillas ( G. beringei ) and chimpanzees ( P. troglodytes ), but not from bonobos ( P. paniscus ) ( Table 1 ). Infections were most common in central chimpanzees ( P. t. troglodytes ) and western lowland gorillas ( G. g. gorilla ), with infected individuals identified at 76% of field sites, including six locations where P. vivax was found in both of these species ( Fig. 1 ). Ape P. vivax was also endemic in eastern chimpanzees ( P. t. schweinfurthii ) and eastern lowland gorillas ( G. b. graueri ), with infected apes documented at 38% of field sites. Despite this wide geographic distribution ( Fig. 1 ), the proportion of ape faecal samples that contained P. vivax -like sequences at any given field site was low: among 2,871 chimpanzee and 1,844 gorilla samples that were analysed, only 45 and 32 were found to be PCR positive, respectively ( Table 1 ). Correcting for specimen degradation and redundant sampling, and taking into account the sensitivity of the non-invasive diagnostic test, we estimated the proportion of P. vivax -sequence-positive individuals for each field site ( Supplementary Table 1 ). The resulting values of 4–8% ( Table 1 ) were lower than prevalence rates previously determined for P. falciparum -like ( Laverania ) parasites in wild apes [10] , but they were very similar to P. vivax parasite rates reported for endemically infected human populations [1] . In humans, point estimates of patent blood infection rarely exceed 7%, even in hyperendemic areas, and a parasite rate of greater than 1% indicates stable transmission [1] . Figure 1: Geographic distribution of P. vivax in wild-living apes. Field sites are shown in relation to the ranges of three subspecies of the common chimpanzee ( P. t. ellioti, magenta; P. t. troglodytes , red; and P. t. schweinfurthii , blue), western ( G. gorilla , yellow) and eastern ( G. beringei , light green) gorillas, as well as bonobos ( P. paniscus , green). Circles, squares and hexagons identify field sites where wild-living chimpanzees, gorillas or both species were sampled, respectively. Ovals indicate bonobo sampling sites. Triangles denote the location of wildlife rescue centres (see Supplementary Table 1 for a list of all field sites and their two-letter codes). Forested areas are shown in dark green, while arid and semiarid areas are depicted in yellow and brown, respectively. Major lakes and major rivers are shown in blue. Dashed white lines indicate national boundaries. Sites where ape P. vivax was detected are highlighted in yellow, with red lettering indicating that both chimpanzees and gorillas were infected. Full size image Table 1 Magnitude of the sylvatic P. vivax reservoir. Full size table Since human P. vivax can induce dormant liver infections, we considered the possibility that ape parasite DNA might be excreted into faeces in the absence of a productive blood-stage infection and thus inflate our infection rate estimates. To examine this, we compared the sensitivity of PCR-based parasite detection in blood and faecal samples from captive chimpanzees housed at a wildlife rescue centre (SY). Importantly, these chimpanzees were kept in outside enclosures immediately adjacent to the habitat of wild apes and were thus exposed to the same mosquito populations. 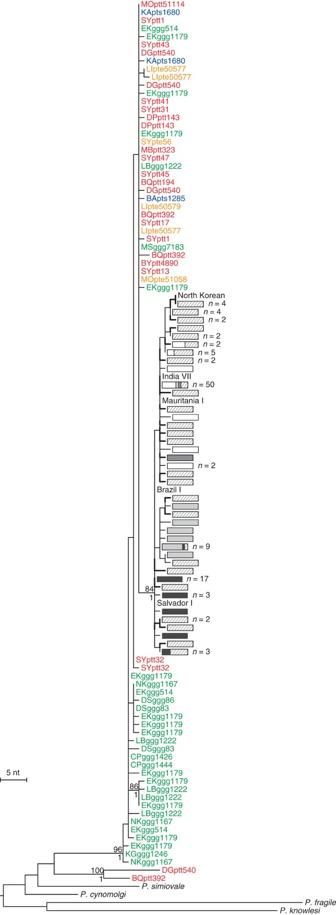Figure 2: Evolutionary relationships of ape and humanP. vivaxparasites in mitochondrial gene regions. The phylogenetic positions of mitochondrial fragment D (2,524 bp;Supplementary Fig. 1a) sequences from ape and humanP. vivaxstrains are shown in relation to human and macaque parasite reference sequences. All sequences were generated by SGA20, except for human (Salvador I, India VII, Mauritania I, North Korean and Brazil I) and simian reference strains from the database (seeSupplementary Tables 6–8for GenBank accession numbers). Ape sequences are colour coded, with capital letters indicating the field site (Fig. 1) and lower case letters denoting species and subspecies origin (ptt:P. t. troglodytes, red; pte:P. t. ellioti, orange; pts:P. t. schweinfurthii, blue; ggg:G. g. gorilla, green). Human sequences are depicted by haplotype (rectangles) and labelled according to their geographic origin in Oceania (light grey), Africa (white), South and Central America (black), South and Southeast Asia (striped) and the Middle East (dark grey). Haplotypes that include more than one sequence are indicated, with the numbers of sequences listed to the right. A second lineage of related parasite sequences from chimpanzee samples DGptt540 and BQptt392 likely represents a newPlasmodiumspecies. The tree was inferred using maximum likelihood methods56. Numbers above and below nodes indicate bootstrap values (≥70%) and Bayesian posterior probabilities (≥0.95), respectively (the scale bar represents five nucleotide substitutions). Although blood and faecal samples were not matched, 11 of 48 chimpanzees (23%) were found to be P. vivax positive by blood analysis, as compared with 1 of 68 chimpanzees (1.5%) by faecal analysis ( Supplementary Table 2 ). Thus, faecal P. vivax detection is considerably less sensitive than blood detection, most probably because of lower parasite loads, and may underestimate the number of infected apes by an order of magnitude. This likely explains our failure to detect ape P. vivax in wild-living Nigeria–Cameroonian chimpanzees ( P. t. ellioti ) and Cross River gorillas ( G. g. diehli ), for which only very few faecal samples were available ( Table 1 ). 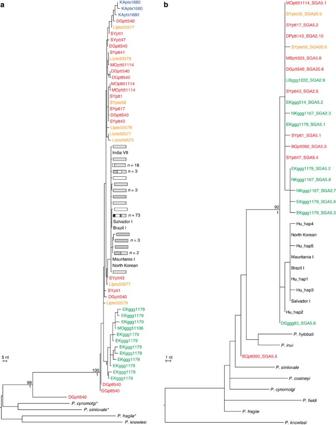Figure 3: Evolutionary relationships of ape and humanP. vivaxparasites in nuclear and apicoplast gene regions. The phylogenetic positions of (a) lactate dehydrogenase (ldh) gene (711 bp) and (b) caseinolytic protease C (clpC) gene (574 bp) sequences from ape and humanP. vivaxstrains are shown in relation to human and macaque parasite reference sequences. All sequences were generated by SGA20, except for human (Salvador I, India VII, Mauritania I, North Korean and Brazil I) and simian reference strains from the database (asterisks indicate SGA-derivedldhsequences forP. simiovale,P. cynomolgiandP. fragile; seeSupplementary Tables 6–8for GenBank accession numbers). Newly derived apeP. vivaxsequences are labelled and colour coded as inFig. 2. Human and simian reference sequences are shown in black. Humanldhhaplotypes are depicted as described inFig. 2. Related parasite sequences from chimpanzee samples DGptt540 (ldh) and BQptt392 (clpC) likely represent a newPlasmodiumspecies. Trees were inferred using maximum likelihood methods56. Numbers above and below nodes indicate bootstrap values (≥70%) and Bayesian posterior probabilities (≥0.95), respectively (the scale bar represents five and one nucleotide (nt) substitutions, respectively). Indeed, we subsequently confirmed P. vivax infection by blood analysis in five Nigeria–Cameroonian chimpanzees that were sampled in captivity ( Supplementary Table 3 ), and although not tested in this study, western chimpanzees ( P. t. verus ) have previously been shown to carry this parasite in the wild [12] . Thus, all four subspecies of the common chimpanzee as well as western and eastern gorillas are infected with P. vivax , indicating the existence of a substantial sylvatic reservoir. Given the widespread infection of both chimpanzee and gorilla populations, the fact that over 700 bonobo faecal samples from eight different collection sites were P. vivax negative came as a surprise ( Fig. 1 ). Since wild-living bonobos also lack P. falciparum -related parasites [10] , yet are susceptible to infection with human P. falciparum in captivity [21] , this finding may reflect a paucity of transmitting mosquito vectors. In humans, a mutation (T to C, at position -33) in the GATA-1 transcription-factor-binding site within the promoter region of the DARC gene [22] yields resistance to P. vivax infection, but sequence analysis of the same region in 134 ape samples, including 28 from bonobos, indicated that none had this substitution ( Supplementary Fig. 2 ). In addition, all ape DARC genes analysed encoded a blood-group antigen with aspartic acid at amino acid 42, rather than the glycine found in the protective Fy a allele in humans ( Supplementary Fig. 2 ) [23] . Finally, we asked whether other primates in central Africa might harbour P. vivax -like parasites. Using the same P. vivax -specific PCR primers, we screened 998 blood samples from 16 Old World monkey species that had previously been collected for molecular epidemiological studies of simian immunodeficiency viruses [24] , [25] . Testing samples from 11 different locations in southern Cameroon and the western parts of the Democratic Republic of the Congo (DRC), we failed to detect P. vivax infection in any of the animals tested ( Supplementary Fig. 3 ). Although 501 of the 998 blood samples (50.2%) yielded a PCR amplicon, all of these represented Hepatocystis spp. infections as determined by sequence analysis ( Supplementary Table 4 ). Thus, we found no evidence for a P. vivax reservoir in these African monkey species. SGA of P. vivax sequences To examine the evolutionary relationships of ape and human parasites, we amplified the complete P. vivax mitochondrial genome in three partially overlapping fragments ( Supplementary Fig. 1a ). This was done using SGA followed by direct amplicon sequencing, which eliminates Taq polymerase-induced recombination and nucleotide substitution errors, and provides a proportional representation of the parasite sequences that are present in vivo [10] , [20] . Alignment of these sequences revealed two single-nucleotide variants (SNVs) that distinguished all ape from all human parasites ( Supplementary Fig. 1b ; a third previously proposed SNV [13] was polymorphic among the ape samples in our dataset). We thus designed PCR primers to amplify a fragment (fragment D) that included both SNVs on the same SGA amplicon ( Supplementary Fig. 1 ). Although only a subset of P. vivax -positive faecal samples yielded this larger mtDNA fragment, we were able to generate fragment D sequences from 22 chimpanzees and 9 gorillas, 17 of which were sampled in the wild ( Supplementary Table 3 ). Since most database sequences are derived by conventional PCR approaches, we also used SGA to amplify fragment D sequences from the blood of P. vivax -infected humans to produce Taq polymerase error-free sequences [20] . These samples included 94 international travellers, who had acquired P. vivax while visiting malaria endemic areas, as well as 25 P. vivax -infected individuals from China, Thailand, Myanmar and India, who sought treatment for clinical malaria ( Supplementary Table 5 ), and thus provide a globally representative sample of human P. vivax infections. Phylogenetic analysis of all SGA-derived P. vivax mtDNA sequences showed that the ape parasites formed two distinct clades ( Fig. 2 ). One clade, represented by sequences from just two chimpanzee samples (termed BQptt392 and DGptt540; see legend of Fig. 2 for an explanation of sample nomenclature), was almost as divergent from the remaining ape and human parasites as were other Plasmodium species, and thus likely represents a previously unidentified species. All other ape parasite sequences were closely related to each other and to human P. vivax sequences, and thus appear to represent a single species ( Fig. 2 ). Within this P. vivax clade, chimpanzee- and gorilla-derived sequences were interspersed, but all human-derived sequences formed a single well-supported lineage that fell within the radiation of the ape parasites. Inclusion of previously published non-SGA sequences confirmed this topology, although many of the database sequences exhibited long branches suggestive of PCR errors ( Supplementary Fig. 4a ). Interestingly, the one P. vivax sequence recently identified in a European traveller who became infected after working in a central African forest [13] did not fall within the human P. vivax lineage, but clustered with parasites obtained from wild-living chimpanzees and gorillas ( Supplementary Fig. 4a ). This confirms the suspicion that this traveller acquired his infection by cross-species transmission from a wild ape. Figure 2: Evolutionary relationships of ape and human P. vivax parasites in mitochondrial gene regions. The phylogenetic positions of mitochondrial fragment D (2,524 bp; Supplementary Fig. 1a ) sequences from ape and human P. vivax strains are shown in relation to human and macaque parasite reference sequences. All sequences were generated by SGA [20] , except for human (Salvador I, India VII, Mauritania I, North Korean and Brazil I) and simian reference strains from the database (see Supplementary Tables 6–8 for GenBank accession numbers). Ape sequences are colour coded, with capital letters indicating the field site ( Fig. 1 ) and lower case letters denoting species and subspecies origin (ptt: P. t. troglodytes , red; pte: P. t. ellioti , orange; pts: P. t. schweinfurthii , blue; ggg: G. g. gorilla , green). Human sequences are depicted by haplotype (rectangles) and labelled according to their geographic origin in Oceania (light grey), Africa (white), South and Central America (black), South and Southeast Asia (striped) and the Middle East (dark grey). Haplotypes that include more than one sequence are indicated, with the numbers of sequences listed to the right. A second lineage of related parasite sequences from chimpanzee samples DGptt540 and BQptt392 likely represents a new Plasmodium species. The tree was inferred using maximum likelihood methods [56] . Numbers above and below nodes indicate bootstrap values (≥70%) and Bayesian posterior probabilities (≥0.95), respectively (the scale bar represents five nucleotide substitutions). Full size image To examine the robustness of these phylogenetic relationships, we selected additional genomic regions that had previously been used for evolutionary studies of P. vivax [7] , [26] . These included portions of the apicoplast caseinolytic protease C ( clpC ) gene as well as the nuclear genes encoding lactate dehydrogenase ( ldh ), adenylosuccinate lyase (asl ), cell division cycle 2-related kinase ( crk2 ) and β -tubulin ( β-tub ). Although fewer ape samples yielded amplification products, this was most likely due to lower copy numbers of apicoplast and nuclear genomes compared with mtDNA. Nonetheless, many samples yielded more than one P. vivax haplotype, indicating coinfection with multiple locally circulating variants ( Supplementary Table 3 ). To increase the number of suitable reference sequences, we also amplified these same fragments from P. vivax -positive human samples, and for some gene regions from related macaque parasites. The resulting phylogenies yielded very similar topologies, with human parasites always forming a monophyletic lineage. Moreover, this lineage fell within the radiation of the P. vivax -like ape sequences for five of the six loci tested ( Fig. 3 ; Supplementary Figs 5–7 ). In contrast, chimpanzee and gorilla sequences were again interspersed, suggesting that P. vivax is often transmitted between the two ape hosts. Figure 3: Evolutionary relationships of ape and human P. vivax parasites in nuclear and apicoplast gene regions. The phylogenetic positions of ( a ) lactate dehydrogenase ( ldh ) gene (711 bp) and ( b ) caseinolytic protease C ( clpC ) gene (574 bp) sequences from ape and human P. vivax strains are shown in relation to human and macaque parasite reference sequences. All sequences were generated by SGA [20] , except for human (Salvador I, India VII, Mauritania I, North Korean and Brazil I) and simian reference strains from the database (asterisks indicate SGA-derived ldh sequences for P. simiovale , P. cynomolgi and P. fragile ; see Supplementary Tables 6–8 for GenBank accession numbers). Newly derived ape P. vivax sequences are labelled and colour coded as in Fig. 2 . Human and simian reference sequences are shown in black. Human ldh haplotypes are depicted as described in Fig. 2 . Related parasite sequences from chimpanzee samples DGptt540 ( ldh ) and BQptt392 ( clpC ) likely represent a new Plasmodium species. Trees were inferred using maximum likelihood methods [56] . Numbers above and below nodes indicate bootstrap values (≥70%) and Bayesian posterior probabilities (≥0.95), respectively (the scale bar represents five and one nucleotide (nt) substitutions, respectively). Full size image The apicoplast and nuclear gene sequences also confirmed the existence of the second, closely related, ape Plasmodium species. Sequences obtained for the clpC , ldh and crk2 genes ( Fig. 3 ; Supplementary Fig. 6 ) from one or the other of the same two chimpanzee samples that yielded divergent mtDNA sequences (DGptt540 and BQptt392) were again clearly distinct from P. vivax . In the mtDNA, ldh and 5′ crk2 phylogenies, this new species was the closest relative of P. vivax (although strong support for this was only found in the latter two trees), while in the other trees relationships were not well resolved. While the new species appears to be rare, it was found in samples from two locations about 110 km apart. Moreover, its detection depended on the cross-reactivity of P. vivax -specific PCR primers, indicating that its prevalence and host association remain to be determined. Nonetheless, existing parasite sequences indicate that African apes harbour not only P. vivax , but also its closest relative. Relative diversity of ape and human P. vivax Since the phylogenetic analyses indicated that human P. vivax strains were derived from within the radiation of ape parasites, we expected the human strains to exhibit lower genetic diversity. To test this directly, we calculated the relative nucleotide diversity of SGA-derived ape and human P. vivax sequences. Indeed, values for the average number of nucleotide differences per site ( π ) were higher for ape parasites than for human parasites at all loci tested. However, the extent of this increased diversity varied among genes ( Table 2 ). For example, the diversity of mtDNA sequences was only 1.4 times higher among the ape parasites than among the human parasites, while for the apicoplast sequence this value was 6 times higher. For nuclear genes the ape sequences were 9 ( asl , ldh ) to 50 ( crk2 ) times more diverse ( Table 2 ). If the levels of diversity were in fact similar in the ape and human parasites, it would be most unlikely to observe this difference consistently across this number of loci (for example, Mann–Whitney U -test applied to the four nuclear loci, P =0.014). Table 2 Nucleotide diversity in human and ape P. vivax lineages. Full size table The relative diversity of the various genes also differed between ape and human parasites. For example, for ape parasites, nuclear gene sequences were 12–25 times more diverse than mtDNA, whereas this ratio was only 1–2 for human parasites ( Table 2 ). In the absence of positive selection or demographic changes, relative diversities within species should be similar to those between species. Thus, for comparison, we calculated distances between orthologous sequences from P. vivax and the closely related P. cynomolgi [9] . For four of the five loci, the relative diversity (scaled to the mtDNA value) among ape P. vivax strains was remarkably similar to the relative interspecific divergence ( Table 2 ); the single exception was crk2 , which was unusually diverse among the ape parasites (compared with other nuclear loci), but also the most conserved nuclear gene between species. In contrast, the diversity values for nuclear and apicoplast genes (relative to mtDNA) among human P. vivax strains were strikingly low ( Table 2 ). This reduced diversity among the human P. vivax strains most likely reflects a recent bottleneck that, depending on the composition of the founder population, could have affected the relative diversity of organelle and nuclear genomes differently. Our finding that wild-living apes in central Africa show widespread infection with diverse strains of P. vivax and harbour a distinct but related Plasmodium species provides new insight into the evolutionary history of human P. vivax , and potentially solves the paradox that a mutation conferring resistance to P. vivax occurs at high frequency in the very region where this parasite is absent. These results indicate that human P. vivax arose from within a Plasmodium species that infects chimpanzees and gorillas and indicate an origin in Africa rather than, as previously assumed, in Asia [6] , [7] , [8] . One interpretation of the phylogenies is that a single host switch from apes gave rise to human P. vivax , analogous to the origin of human P. falciparum [10] . However, this seems unlikely in this case since ape P. vivax does not divide into gorilla- and chimpanzee-specific lineages and since humans are susceptible to both natural [13] and experimental [27] ape P. vivax infections. Thus, a more plausible interpretation is that an ancestral P. vivax stock was able to infect humans, gorillas and chimpanzees in Africa until the Duffy-negative mutation started to spread (perhaps around 30,000 years ago [28] ) and eliminated P. vivax from humans there. Under this scenario, extant human-infecting P. vivax represents a bottlenecked lineage that survived after spreading out of Africa. Much more recently, concomitant with host migrations, human P. vivax has been reintroduced to Africa [29] . Several alternative scenarios for the origins of ape and human P. vivax have recently been discussed [13] , but none of these seems plausible in light of the present data. All previous models assumed that P. vivax originated in humans in Asia, following the cross-species transmission of a monkey parasite, and that humans then brought the parasite to African apes. This assumption has been based on the fact that the closest known relatives of P. vivax all seem to infect Asian primates [6] , [7] , [8] , [9] . However, we now show that chimpanzees harbour a Plasmodium species that is more closely related to P. vivax than are any of the Asian primate parasites. Thus, it is more parsimonious to assume that the common ancestor of these two species existed in Africa. How this lineage was introduced into African apes remains unknown; however, this appears to have occurred a long time before the origin of P. vivax . To explain current levels of genetic diversity in ape and human P. vivax strains, previous models invoking an Asian origin either require human P. vivax in Asia to have gone extinct, prior to repopulation from Africa, or necessitate Asian P. vivax to have gone through a bottleneck (of unknown cause) [13] . In contrast, the African origin model does not require such an ancestral (now extinct) human P. vivax population in Asia, but explains the reduced diversity of human parasites, as resulting from an out-of-Africa bottleneck as seen in P. falciparum [30] , and in humans themselves [31] . It has also been suggested that P. vivax is more likely to have spread from Asia to Africa, because human P. vivax strains in Asia seem to be the most diverse [13] , [32] and because phylogeographic analyses indicated elevated migration rates from Asia (especially India) to Africa [6] . However, this is now explained more simply by the extinction of human P. vivax in Africa, which would have had high diversity, due to the spread of the Duffy-negative mutation. P. vivax strains currently infecting humans in Africa are indeed of Asian origin, but this reflects a reintroduction and occurred only recently, perhaps with the peopling of Madagascar from Asia within the last few thousand years [33] . If the origin of P. vivax had been due to transmission from macaques in southeast Asia, this would imply a convoluted evolutionary history, given the timescales that have been invoked. Estimates of the time of the last common ancestor of human P. vivax are generally on the order of hundreds of thousands of years ago. For example, using mtDNA sequences this ancestor was estimated to have existed about 400,000 years ago [32] , and a more recent comparison of nuclear genome sequences suggested a similar date [34] . Modern humans are thought to have evolved in Africa and to first have entered Asia no more than 60,000 years ago [35] . Thus, if the estimates of the timescale of the coalescence of human P. vivax lineages are correct, the recipient of the transmission from macaques must have been some earlier hominin species, and P. vivax must have diversified for a long time in that host before numerous lineages were transmitted to modern humans after they emerged from Africa. The existence of a sylvatic P. vivax reservoir has public health implications. First, it solves the mystery of P. vivax infections in travellers returning from regions where 99% of the human population is Duffy negative [36] , [37] . Second, it raises the possibility that humans living in close proximity of chimpanzees and gorillas may become infected by ape P. vivax . A recent study of individuals attending a health clinic in the Republic of Congo revealed that 10% carried antibodies specific for preerythrocytic stages of P. vivax , suggesting continuing exposure to P. vivax sporozoites from an unidentified source [38] . Since ape P. vivax is highly prevalent, especially in west central Africa, wild-living chimpanzees and gorillas could serve as an infection reservoir, especially in areas where an influx of Duffy-positive humans through commerce and travel coincides with increasing forest encroachment and ape habitat destruction. Although Duffy-negative individuals are generally protected from blood-stage infections, recent studies in Madagascar [39] and Ethiopia [40] have shown that P. vivax is not absolutely dependent on the Duffy receptor. It will thus be important to assess the potential of ape parasites to acquire this phenotype, once the underlying genetic determinants have been identified in human strains. The possibility that ape P. vivax may spread via international travel to countries where human P. vivax is actively transmitted should also be considered. Since ape P. vivax is much more diverse than human P. vivax ( Figs 2 and 3 ; Table 2 ), it is potentially more versatile to escape treatment and prevention measures, especially if human and ape parasites were able to recombine. Given the documented propensity of P. vivax for host switching [13] , [27] , it seems important to screen Duffy-positive and -negative humans in west central Africa, as well as transmitting mosquito vectors, for the presence of ape P. vivax . Such studies are now possible through the development of molecular tools that distinguish ape from human P. vivax , which also permit the screening of faecal samples for liver-derived parasite DNA in the absence of patent blood infection. These results are necessary to inform malaria control and eradication efforts and to assess future human zoonotic risk. Ape samples A total of 5,469 faecal samples newly (TL site) or previously collected from wild-living chimpanzees ( P. troglodytes ), western gorillas ( G. gorilla ), eastern gorillas ( G. beringei ) and bonobos ( P. paniscus ) for molecular epidemiological studies of simian retroviruses [18] , [19] , [41] , [42] , [43] , [44] and Laverania parasites [10] were selected for P. vivax screening. All specimens were derived from non-habituated apes, except for 170 samples from chimpanzees in Gombe National Park (GM), Tanzania, and 26 samples from gorillas in the Dzanga-Sangha Reserve (DS), Central African Republic, who were habituated to the presence of human observers. Samples were collected (1:1 vol/vol) in RNA later (Life Technologies), transported at ambient temperatures and stored at −80 °C. Faecal DNA was extracted using the QIAamp Stool DNA Mini Kit (Qiagen, Valencia, CA) and used to amplify portions of the host mitochondrial genome to confirm species and subspecies origin [18] , [19] , [41] , [42] , [43] , [44] . A subset was also subjected to microsatellite analysis at 4–8 polymorphic loci [10] , [18] , [41] , [42] , [43] , [44] to estimate the number of sampled individuals ( Supplementary Table 1 ). In addition to faecal samples from wild populations, we also obtained stool and blood samples from sanctuary chimpanzees and gorillas that were kept in outside enclosures immediately adjacent to the habitat of wild apes. These included 113 faecal and 66 blood samples from chimpanzees housed at the Sanaga Yong Rescue Centre (SY), 2 faecal samples from gorillas and 14 blood samples from chimpanzees housed at the Limbe Wildlife Centre (LI) and 8 blood samples from 6 chimpanzees and 2 gorillas housed at the Mfou National Park Wildlife Rescue Centre (MO), all located in Cameroon. Faecal samples were collected from known individuals under direct observation. Blood samples were obtained by veni-puncture (dried blood spots, whole blood, buffy coats, red blood cells) and represented left-over material from routine health examinations or were collected for specific veterinary (diagnostic) purposes. Blood and faecal collections were approved by the Ministry of Forestry and Wildlife of Cameroon. Two chimpanzees at the SY sanctuary were suspected to suffer from malaria and sampled during severe febrile illnesses. One had positive blood smears on site and was subsequently identified to be PCR positive for P. reichenowi , while the other was PCR positive for ape P. vivax . Both responded to malaria treatment. A few additional chimpanzees who were PCR positive for either Laverania or ape P. vivax exhibited milder symptoms at or near the time of sampling, but the majority of captive apes, including several who were Laverania and/or non- Laverania sequence positive by blood analysis, were asymptomatic at the time of blood collection. These individuals were also blood smear negative. Samples were shipped in compliance with Convention on International Trade in Endangered Species of Wild Fauna and Flora regulations and country specific import and export permits. DNA was extracted from whole blood and dried blood spots using the QIAamp Blood DNA Mini Kit (Qiagen, Valencia, CA). Monkey samples To investigate the full host range of P. vivax , we screened blood samples from 998 non-human primates sampled in Cameroon and the Democratic Republic of the Congo ( Supplementary Table 4 ). Collection and molecular characterization of these samples have been described [24] , [25] , [45] , except for samples from the BO, MO, MA and MS field sites ( Supplementary Fig. 3 ). Briefly, samples were collected from primate bushmeat as dried blood spots or whole blood using strategies specifically designed not to increase demand [24] , [25] , [45] . DNA was extracted using the QIAamp blood kit (Qiagen, Courtaboeuf, France) and the species origin was determined by amplifying a 386 bp mtDNA fragment spanning the 12S rRNA gene using single round PCR [24] , [25] . The non-human primate samples were obtained with approval from the Ministries of Health and Environment and the National Ethics Committees of Cameroon and the Democratic Republic of the Congo. Human samples To increase the number of human P. vivax reference sequences and to generate sequences devoid of PCR error, we obtained a global sampling of human P. vivax infections. These included dried blood spots or DNA samples from (i) 61 international travellers diagnosed at the Malaria Reference Laboratory of the London School of Hygiene and Tropical Medicine, London, UK (designated MRL), (ii) 35 international travellers diagnosed at the Department of Infectious Diseases, Karolinska University Hospital, Stockholm, Sweden (designated SW), and (iii) 32 residents of malaria endemic areas in China (designated GX; n =10), Myanmar (V0; n =10), Thailand (PVAR; n =2) and India (IN; n =10), who sought treatment at local health clinics ( Supplementary Table 5 ). In all cases, P. vivax infection was initially identified by microscopy and then confirmed by diagnostic PCR followed by direct amplicon sequencing. DNA was extracted from whole blood or dried blood spots using QIAamp DNA Mini Kit (Qiagen, Valencia, CA). Anonymised DNA samples previously collected by the MRL were provided under its remit to undertake epidemiological surveillance relevant to imported malaria in the UK. All other subjects provided written informed consent for the collection and analysis of samples, which were sent without patient identifiers and other patient information, except for the country of (known or presumed) P. vivax acquisition. The study was approved by the Institutional Review Boards of the University of Pennsylvania, the Karolinska Institute and the Pennsylvania State University. Other Plasmodium species Genomic DNA from, or dried blood spots containing, P. inui (catalogue number MRA-486F), P. simiovale (MRA-488F), P. cynomolgi (MRA-350G) and P. fragile (MRA-352G) were obtained from the Malaria Research and Reference Reagent Resource Center (MR4) of the American Type Culture Collection (ATCC, Manassas, VA) to generate single-genome-derived reference sequences for phylogenetic analyses. Microsatellite analyses Ape faecal samples that have previously been subjected to microsatellite analyses have been reported [10] , except for bonobo samples obtained at the TL field site, which were obtained more recently. Briefly, faecal DNA was extracted and used to amplify eight polymorphic microsatellite loci. Amplification products were analysed on an automated sequencer (Applied Biosystems, CA) and sized using GeneMapper 4.0 (Applied Biosystems). For individual identification, samples were first grouped by mtDNA haplotype. Within each haplotype, samples were then grouped by microsatellite genotypes. Since samples were partially degraded due to prolonged storage at ambient temperatures, we allowed allelic mismatches at up to six loci to guard against allelic dropout, but only if they represented a missing allele. This conservative genotyping approach likely underestimates the number of individuals screened and thus reflects a minimum estimate. Samples with evidence of DNA admixture (multiple peaks for the same locus) were discarded. P. vivax diagnostic PCR Faecal and blood samples were screened by conventional PCR for P. vivax mitochondrial ( cox1 ) sequences as described [46] . Although originally designed to amplify P. vivax sequences from samples coinfected with Laverania species, the primers were also found to amplify Hepatocystis spp. mtDNA ( Supplementary Table 4 ). Primers Pv2768p (5′-GTATGGATCGAATCTTACTTATTC-3′) and Pv3287n (5′-AATACCAGATACTAAAAGACCAACAATGATA-3′) were used in the first round of PCR, while Pv2870p (5′-TTGCAATCATAAAACTTTAGGTC-3′) and Pv3185n (5′-TCCTCCAAATTCTGCTGCTGTAGATAAAATG-3′) were used in the second round, yielding a 297 bp amplicon ( Supplementary Fig. 1a ). Amplicons were gel purified and sequenced directly to confirm Plasmodium infection. SGA of P. vivax gene sequences To derive P. vivax sequences devoid of PCR errors, including Taq polymerase-induced misincorporations and template switching, blood and faecal samples from P. vivax -infected apes and humans were subjected to SGA methods, essentially as described [10] , [20] . DNA was extracted and end point diluted such that fewer than 30% of PCR reactions yielded an amplification product. According to a Poisson distribution, a well yielding a PCR product at this dilution will contain only a single amplifiable template more than 83% of the time. Multiple different gene regions were amplified, including mitochondrial fragments S, A, B, C and D ( Supplementary Fig. 1a ), the apicoplast clpC gene (574 bp), and the nuclear genes ldh (713–724 bp), asl (838 bp), crk 2 (666 bp) and β-tub (684 bp) ( Supplementary Table 3 ). Primers were designed in conserved regions of the P. vivax genome, except for a set of ldh primers intended to amplify more diverse macaque parasites, which were designed using both P. vivax and P. knowlesi consensus sequences ( Supplementary Table 9 ). PCR cycling conditions were as described [10] , except for varying elongation times depending on the length of the amplicon (1min per 1 kb amplicon length). Amplification products were sequenced directly and analysed using Sequencher (Gene Codes Corporation, Ann Arbor, MI). All sequences with double peaks in the chromatogram were discarded, except for sequences derived from ape faecal samples that contained a single double peak. Single double peaks in SGA sequences either indicate the presence of two P. vivax variants differing by a single nucleotide or a PCR misincorporation within the first or second round of PCR. We resolved these ambiguous sites by selecting the nucleotide that was identical to the ape P. vivax consensus. This conservative approach avoided the loss of otherwise valuable sequence information. GenBank accession codes of newly derived SGA sequences are listed in Supplementary Tables 6 and 7 . DARC genotyping To examine whether P. vivax -infected and -uninfected apes exhibited sequence polymorphisms in their DARC promoter and/or adjacent coding sequences, we amplified a 1,286 bp region of the DARC gene in two partially overlapping PCR fragments from 134 ape (faecal and blood) samples ( Supplementary Fig. 2a ). Fragment A was amplified using DARCpF1 (5′-GCTGTCCCATTGTCCCCTAG-3′) and DARCpR8 (5′-GGCCCCATACTCACCCTGTGC-3′) in the first round of PCR, and DARCpF3 (5′-GCACAATGATACACAGCAAAC-3′) and FYPdn (5′-CCATGGCACCGTTTGGTTCAGG-3′) [47] in the second round. Fragment B was amplified using DARC_F5 (5′-AGGCAGTGGGCGTGGGGTAAG-3′) and DARC_R5 (5′-AGCCATACCAGACACAGTAGCC-3′) in the first round, and DARC_NTF1 (5′-TTGGCTCTTATCTTGGAAGCAC-3′) and DARC_NTR1 (5′->TGGTGAGGATGAAGAAGGGCAGT-3′) in the second round. PCR conditions were the same as those used to amplify P. vivax mtDNA. Amplicons were directly sequenced and analysed using Sequencher. Ape P. vivax infection rates For sites where the number of sampled chimpanzees was known ( Supplementary Table 1 ), P. vivax infection rates were estimated based on the proportion of positive individuals (but correcting for test sensitivity; see below), with 95% confidence limits determined assuming binomial sampling. For field sites where the number of sampled individuals was not known, infection rates were estimated based on the number of faecal samples, but correcting for specimen degradation, oversampling and the sensitivity of the diagnostic PCR test. The latter was estimated by determining the proportion of PCR-positive specimens from P. vivax -infected apes that were sampled more than once on the same day, as previously described [10] . Including data from 14 such apes (6 central chimpanzees, 5 eastern chimpanzees and 3 western gorillas), we estimated the sensitivity to be 32% (17 of 53 samples were positive; confidence limits were determined assuming binomial sampling). Using previously reported values for oversampling [10] (1.77, 1.84, 3.74, 2.06 and 1.84 for central chimpanzees, western gorillas, eastern chimpanzees, eastern gorillas and bonobos, respectively) and sample degradation [10] (0.13), the proportion of P. vivax -sequence-positive apes was estimated for each field site ( Table 1 and Supplementary Table 1 ). However, since P. vivax detection in faecal samples is considerably less sensitive than in blood, the resulting prevalence rates should be interpreted as minimum estimates. Nucleotide diversity calculations Newly generated ape and human P. vivax sequences were aligned with sequences from the complete genomes of five P. vivax reference strains (Salvador I, India VII, Mauritania I, North Korean and Brazil I). Other than these five reference strains, only SGA-derived sequences were included in the analysis, so as to not inflate diversity values by including Taq polymerase-induced errors. Identical sequences from the same sample or individual were excluded; identical sequences from different samples or individuals were retained. For each gene, sequences were aligned using ClustalW [48] , and both ape and human P. vivax alignments were trimmed to the same length. The nucleotide diversity ( π ) of human and ape parasite sequences was calculated for six P. vivax gene fragments (mtDNA fragment D, apicoplast clpC , nuclear ldh , asl , crk2 and β-tub ) using DnaSP version 5.10 (ref. 49 ). Distance calculation from P. cynomolgi For each P. vivax gene, the same set of sequences as used for the diversity calculation was aligned with one P. cynomolgi reference sequence [9] . The distance from each P. vivax sequence to the P. cynomolgi reference was calculated using the R package version 3.0–8 with the Tamura–Nei correction [50] , [51] , and the mean distance was calculated for each gene. Phylogenetic analyses Sequence alignments were constructed using ClustalW version 2.1 (ref. 48 ) and manually adjusted using MacClade [52] . Regions that could not be unambiguously aligned were omitted from subsequent phylogenetic analyses. Nuclear gene sequences were subjected to recombination analysis using GARD [53] . Evolutionary models for phylogenetic analyses were determined using the Akaike information criterion with Modeltest (version 3.7) [54] and PAUP* (ref. 55 ). Maximum likelihood phylogenies with bootstrap support (100 replicates) were estimated jointly with model parameter values by means of PhyML (version 3) [56] using both nearest-neighbour interchange and subtree pruning and regrafting with Neighbor Joining and 10 random-addition starting trees [57] . Posterior probabilities for nodes in phylogenetic trees were calculated using MrBayes (version 3.2) [58] , using an average standard deviation of partition frequencies <0.01 as a convergence diagnostic. Trees were constructed from mitochondrial fragment D sequences (2,524 bp, Fig. 2 and Supplementary Fig. 4a ), apicoplast clpC sequences (574 bp, Fig. 3b ), and nuclear β-tub (664 bp, Supplementary Fig. 5 ), ldh (711 bp, Fig. 3a and Supplementary Fig. 4b ), crk2 (271 and 372 bp, Supplementary Fig. 6 ) and asl (838 bp, Supplementary Fig. 7 ) sequences. Accession codes: All newly derived ape and human Plasmodium sequences have been deposited in the GenBank Nucleotide Sequence Database under accession codes KF591752 — KF591851 and KF618374 — KF618618 , respectively. DARC sequences have been deposited in the GenBank Nucleotide Sequence Database under accession codes KF618448 — KF618495 . How to cite this article: Liu, W. et al. African origin of the malaria parasite Plasmodium vivax . Nat. Commun. 5:3346 doi: 10.1038/ncomms4346 (2014).